Magnetic behaviour of TbPc2single-molecule magnets chemically grafted on silicon surface Single-molecule magnets (SMMs) are among the most promising molecular systems for the development of novel molecular electronics based on spin transport. Going beyond investigations focused on physisorbed SMMs, in this work the robust grafting of terbium(III) bis(phthalocyaninato) complexes to a silicon surface from a diluted solution is achieved by rational chemical design yielding the formation of a partially oriented monolayer on the conducting substrate. Here by exploiting the surface sensitivity of X-ray circular magnetic dichroism, we evidence an enhancement of the magnetic bistability of this SMM, in contrast to the dramatic reduction of the magnetic hysteresis that characterizes monolayer deposits evaporated on noble and ferromagnetic metals. Photoelectron spectroscopy investigations and density functional theory analysis suggest a non-innocent role played by the silicon substrate, evidencing the potentiality of this approach for robust integration of bistable magnetic molecules in electronic devices. Molecular-based functional materials can allow the exploitation of the richness of molecular structures to implement in technology novel and unexpected properties. Among the next-generation sensors, transistors and memory devices, those based on spin state of molecules represent promising alternatives to traditional technologies [1] , [2] . In this context, there is a keen interest on single-molecule magnets (SMMs) [3] , functional molecules featuring magnetic memory at the single-molecule scale [4] , [5] and quantum effects [6] , [7] , [8] , [9] . However, beyond temperature limitations, a quick development of a SMM-based technology is hampered by the intrinsic chemical fragility of most polynuclear SMMs and the evanescence of the SMM behaviour, which make the retention of the molecular magnetic bistability at the nanoscale far from trivial. The chemical bond between a sulphur-functionalized tetrairon(III) SMM, Fe 4 and a gold surface has been recently employed and the typical magnetic hysteresis observed through synchrotron light-based experiments [10] , [11] . However, the lability of the Au–S bond [12] cannot guarantee the long-term stability required for the development of an SMM-based device. For this reason, grafting of SMMs on a particularly attractive inorganic platform such as silicon wafers offers the possibility to make robust and durable devices by forming stable Si–C covalent bonds. Moreover, the possibility of different doping of the silicon substrate can be used to influence the electronic properties of the grafted molecules [13] and the mobility of the charge carriers in the final hybrid device. Although preliminary promising results have been obtained with Fe 4 SMMs chemically anchored on silicon [14] , the very low temperature required for the observation of magnetic bistability (below 1 K) has prompted us to another molecule, that is the terbium(III) bis(phthalocyaninato) neutral complex [15] , TbPc 2 hereafter. Slow dynamics in the magnetization reversal is here due to the large activation energy barrier generated by crystal field splitting of the J =6 ground multiplet of the highly anisotropic Tb III ion [16] . This results in one of the most promising and widely investigated SMMs [17] , [18] , [19] , [20] , [21] , [22] , the insertion of which in single-molecule transport devices has allowed to monitor the quantum dynamics of a single-nuclear spin [23] and to observe a novel supramolecular spin valve effect [24] . In general, however, the magnetization dynamics of TbPc 2 is severely altered in amorphous materials, where the packing of the molecules characterizing the crystalline phase is lost [25] , [26] . The origin of the phenomenon remains unclear, although it should be considered that small distortion of the two phthalocyaninato ligands from the perfectly staggered configuration, corresponding to D 4d symmetry, can be very efficient in promoting the tunnel mechanism of relaxation [26] . A similar reduction of the magnetic bistability is observed at the nanoscale: by thermal evaporation of these double-deckers on clean metallic surfaces in ultra-high-vacuum (UHV) environment, the wide opening of the magnetic hysteresis loop above liquid helium temperature vanishes [27] , [28] . The phthalocyaninato ligands appear to efficiently couple the magnetic moment of the Tb ion with the magnetization of substrates as recently shown for submonolayer UHV-prepared deposits of TbPc 2 on magnetic substrates [29] , [30] . The strength of the interaction can be tuned by modifying the electronic characteristics of the substrate, although also in these cases no evidence of the SMM character of the pristine molecular system has been observed. Here we report the outcome of an alternative approach aimed at the exploitation of the magnetic bistability of double-decker systems in a robust nanostructure, prerequisite to fruitfully benefit from SMM features in ad hoc designed molecular devices. This has been achieved by the functionalization of the original TbPc 2 system, resulting in a homoleptic double-decker derivative bearing long aliphatic chains with terminal double bonds that allow the grafting of the molecule to the silicon surface from a diluted solution. By using X-ray Circular Magnetic Dichroism to extract the magnetic properties at the nanoscale with the support of other parallel chemical and structural characterizations flanked by theoretical analysis, we demonstrate that SMM behaviour with enhanced hysteresis is retained on a partially ordered and chemically robust monolayer of molecules grafted on Si(100) surface through hydrosilylation reaction. Synthesis of the TbPc 2 (OC 11 H 21 ) 8 complex Silicon was chosen as surface for grafting because of its technological relevance and for the possibility to form thermally and hydrolytically stable Si–C bonds via thermal hydrosilylation [31] . The design of a suitable TbPc 2 for silicon grafting requires the introduction of ω-functionalized alkyl chains at peripheral positions of the phthalocyanine ligands. The classical De Cian synthesis [32] , starting from the terbium(III) acetylacetonate and 1,2-dicyanobenzene derivatives, has been adopted here. The alternative option of TbPc 2 post-functionalization turned out to be synthetically unfeasible in this case. Moreover, the only substituents compatible with the harsh reaction conditions required for double-decker formation were alkoxy derivatives, excluding most of the common linker groups such as esters, amides and carbamates. The required 4-(ω-undecenyloxy)phthalonitrile precursor [33] was synthesized from the commercially available 4-hydroxyphthalonitrile by the addition of 11-bromo-1-undecene in the presence of an excess of potassium carbonate in dimethylformamide in 80% yield. Homoleptic TbPc 2 (OC 11 H 21 ) 8 was then obtained by heating terbium(III) acetylacetonate in refluxing 1-hexanol in the presence of 4-(ω-undecenyloxy)phthalonitrile, with 1,8-diazabicyclo[5.4.0]undec-7-ene as a basic catalyst ( Fig. 1a ). The neutral double-decker compound was isolated in 35% yield as a mixture of constitutional isomers in the form of dark-green powder (see Methods and Supplementary Note 1 ). 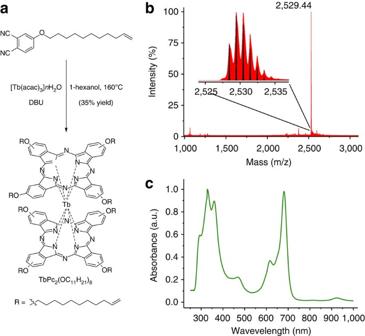Figure 1: Synthesis and chemical characterization of TbPc2(OC11H21)8. (a) Synthesis of homoleptic TbPc2(OC11H21)8using 4-(ω-undecenyloxy)phthalonitrile as starting material. (b) High-resolution MALDI-TOF spectrum of TbPc2(OC11H21)8, with experimental (red lines) versus theoretical (black) isotopic distribution pattern in the inset. (c) Ultraviolet–visible absorption spectrum of TbPc2(OC11H21)8in chloroform. Figure 1: Synthesis and chemical characterization of TbPc 2 (OC 11 H 21 ) 8 . ( a ) Synthesis of homoleptic TbPc 2 (OC 11 H 21 ) 8 using 4-(ω-undecenyloxy)phthalonitrile as starting material. ( b ) High-resolution MALDI-TOF spectrum of TbPc 2 (OC 11 H 21 ) 8 , with experimental (red lines) versus theoretical (black) isotopic distribution pattern in the inset. ( c ) Ultraviolet–visible absorption spectrum of TbPc 2 (OC 11 H 21 ) 8 in chloroform. Full size image The resulting TbPc 2 (OC 11 H 21 ) 8 was characterized via high-resolution matrix-assisted laser desorption ionization–time-of-flight (MALDI-TOF) mass spectrometry, X-ray photoelectron spectroscopy (XPS) and ultraviolet–visible spectroscopy (see Fig. 1 and Supplementary Note 2 ). Mass spectrometry, the most employed analytical tool for this class of compounds, revealed a unique peak centred at 2,529.44 m / z that corresponds well in position and isotopic distribution to the calculated ones for the molecular ion of TbPc 2 (OC 11 H 21 ) 8 ( Fig. 1b and inset). The ultraviolet–visible spectrum of TbPc 2 (OC 11 H 21 ) 8 recorded in chloroform solution shown in Fig. 1c confirms the neutral π radical form of the molecule: the spectrum exhibits the characteristic absorption bands of double-decker phthalocyaninato complexes [34] . The Q band at 681 nm results from the promotion of an electron from the first semi-occupied molecular orbital to the second lowest unoccupated molecular orbital (LUMO) and from the second fully occupied highest occupated molecular orbital (HOMO) to the first LUMO. Furthermore, the spectrum shows a typical split Soret-band, resulting from the electronic transitions from the third occupied HOMO to the first LUMO, with maxima at 329 and 361 nm. The two weak π-radical bands at 469 and 926 nm are due to electronic transitions from the semi-occupied molecular orbital orbital to the degenerate LUMOs. The multiplicity associated to the several isomers of TbPc 2 (OC 11 H 21 ) 8 produced in the reaction does not allow the univocal attribution of all resonances by nuclear magnetic resonance ( Supplementary Fig. 1 ). However, the strong paramagnetic upfield shifts at negative p.p.m. are indicative of Tb complexation even if the presence of these paramagnetic units hampers a proper spectral assignment of the aromatic protons. XPS spectra of a reference bulk phase have been recorded on a thick film prepared by drop casting a diluted dichloromethane solution of the complexes on a polycrystalline gold substrate. A semi-quantitative analysis of the spectra ( Supplementary Fig. 2 and Supplementary Table 1 ) reveals an atomic composition of the compound in agreement, within the limits of the technique, with the proposed formula, thus confirming the mass spectrometry results. Magnetic characterization of bulk TbPc 2 (OC 11 H 21 ) 8 Magnetic characterization, performed with standard a.c. and d.c. magnetometric techniques ( Fig. 2 , Supplementary Fig. 3 ), clearly indicates the SMM behaviour of the complex in its bulk phase. In zero static field, the a.c. susceptibility versus temperature curves are characterized by a frequency-dependent peak in the out-of-phase component occurring at relatively high temperatures, for example, the maximum in χ ′′ at 1 kHz is observed at 47 K, which well compares with those reported for similar homoleptic substituted TbPc 2 systems [35] . A more careful analysis of the frequency dependence of the a.c. susceptibility in a wide-frequency range, 0.5 Hz–10 kHz, was performed with the extended Debye model [3] allowing to extract the relaxation time, τ , and its distribution width through the empirical parameter, α ( Supplementary Note 3 ). The temperature dependence of τ is shown in Fig. 2b . A linear behaviour in the ln( τ ) versus 1/ T plot is observed at zero static field in the high-temperature regime, T >35 K, providing the parameters τ 0 =5.5±0.7 × 10 −12 s and Δ/ k B =811±5 K for the best fit with the Arrhenius law, τ = τ 0 exp(Δ/ k B T ). The estimated energy barrier in the thermally activated process is smaller than that found for the crystalline phase of TbPc 2 (965 K) [35] , but it is close to the value observed in similar conditions for amorphous unfunctionalized TbPc 2 system (856 K) [26] , in agreement with the amorphous character of TbPc 2 (OC 11 H 21 ) 8 sample. Below 35 K, the relaxation becomes temperature independent, indicating the onset of a tunnel mechanism of relaxation, with a significant increase of the width of the distribution of the relaxation times. A better simulation of χ ′′ versus ν curves is achieved taking into account the presence of a bimodal distribution, see Supplementary Fig. 4 , only the dominating one being reported in Fig. 2b . 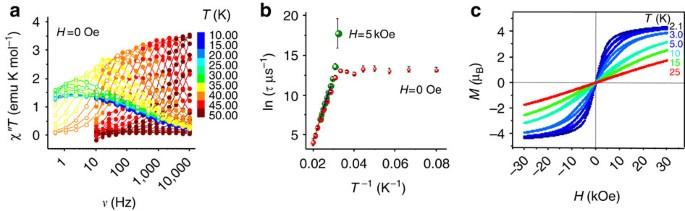Figure 2: Bulk magnetic properties of TbPc2(OC11H21)8. (a) a.c. susceptibility measurements in zero field. (b) Arrhenius plot of data extracted from a.c. measurements in zero field and in a 5-kOe static field. (c) Magnetization curves as a function of the temperature recorded at a field sweeping rate of 50 Oe s−1. Figure 2: Bulk magnetic properties of TbPc 2 (OC 11 H 21 ) 8 . ( a ) a.c. susceptibility measurements in zero field. ( b ) Arrhenius plot of data extracted from a.c. measurements in zero field and in a 5-kOe static field. ( c ) Magnetization curves as a function of the temperature recorded at a field sweeping rate of 50 Oe s −1 . Full size image The application of a static field of 5 kOe (data in Supplementary Figs 3 and 5 ) provides comparable high-temperature behaviour as shown in Fig. 2b , but significantly affects the magnetic relaxation below 35 K, suppressing the tunnelling mechanism with τ exceeding the accessible timescale of the a.c. susceptometer (~10 s). A single distribution of τ is observed in static field because distortions from idealized D 4d symmetry present in this amorphous material are less relevant when resonant quantum tunnelling is suppressed. Magnetization versus field measurements performed at several temperatures and scanning the field between 30 and −30 kOe at 50 Oe s −1 (see Fig. 2c ) evidence the opening of a hysteresis below 15 K with the typical butterfly shape induced by the enhancement of quantum tunnelling in zero applied field [36] . Monolayer preparation and chemical characterization The TbPc 2 (OC 11 H 21 ) 8 complex has been anchored on a H-terminated Si(100) surface via thermal hydrosilylation of the double bonds according to the published literature [37] . The hydrosilylation reaction leads to the formation of a robust Si–C bond and it occurs by placing the alkene-functionalized molecules in a 10 −3 M mesitylene solution at 200 °C in the presence of a freshly etched H-terminated Si(100). After grafting, several cycles of cleaning (including the sonication of the sample in several solvents) guarantee the removal of all the physisorbed materials leaving on the surface only the monolayer of grafted molecules. The silicon-anchored complex, TbPc 2 (OC 11 H 21 ) 8 @Si hereafter, has been characterized by XPS in order to verify the chemical integrity of the system (see Supplementary Note 4 ); only Tb 3d 3/2 , N 1s and C 1s signals have been included in a semiquantitative estimation of the element content on surface and are reported in Supplementary Information (see Supplementary Fig. 2 and Supplementary Table 1 ). Even considering the experimental error of XPS and the presence of adventitious carbon contamination in this ex situ prepared sample, we can assert that the procedure of grafting assures the deposition of the intact system. Additional information on the monolayer nature can be obtained by the analysis of the N 1s peak shape. The comparison between the spectra of the monolayer and that of the thick film, reported in Fig. 3 , evidences in fact significant differences. The drop cast film features a unique peak at 398.3 eV arising from the superposition of the contributions from the pyrrole-aza coordinating the metal and from the meso-bridging aza nitrogen atoms, as expected for a metal coordinated phthalocyanine [38] . On the contrary the N 1s spectral region of the monolayer presents, in addition to this signal, a more intense component at higher energy (400.3 eV), clearly indicating that a modification occurs in the chemisorbed molecules. 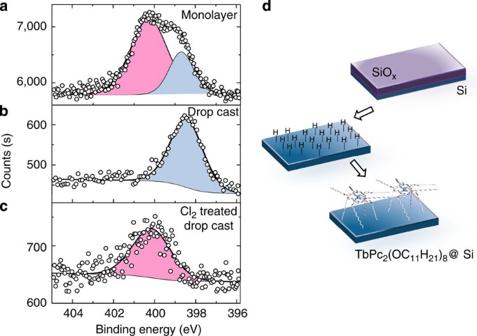Figure 3: Grafting of TbPc2(OC11H21)8. High-resolution N1sXPS spectra of (a) the TbPc2(OC11H21)8@Si monolayer, (b) the drop cast deposit TbPc2(OC11H21)8and (c) the drop cast sample treated with chlorine. (d) Sketch of the TbPc2(OC11H21)8@Si grafting procedure: step (1) etching in 1.0% hydrofluoric acid of silicon surface; step (2) hydrosilylation at 200 °C for 2 h. Figure 3: Grafting of TbPc 2 (OC 11 H 21 ) 8 . High-resolution N 1s XPS spectra of ( a ) the TbPc 2 (OC 11 H 21 ) 8 @Si monolayer, ( b ) the drop cast deposit TbPc 2 (OC 11 H 21 ) 8 and ( c ) the drop cast sample treated with chlorine. ( d ) Sketch of the TbPc 2 (OC 11 H 21 ) 8 @Si grafting procedure: step (1) etching in 1.0% hydrofluoric acid of silicon surface; step (2) hydrosilylation at 200 °C for 2 h. Full size image Interestingly, we show in Fig. 3c that a similar shift to higher energy of the N 1s signal can be induced also on a bulk sample of TbPc 2 (OC 11 H 21 ) 8 by exposing its solution to chlorine and then preparing a drop cast deposit. The treatment with chlorine, already described in literature for Lutetium(III) bis(phthalocyaninato) exposed to Cl 2 under high-vacuum condition [39] , induces the formation of the corresponding cationic double-decker species [40] , that is the oxidized complex in which one of the electrons of the bis(phthalocyaninato) ligands shell has been removed. The fact that this is a surface-induced effect is evidenced by experiments where the TbPc 2 (OC 11 H 21 ) 8 concentration in the solution grafting was reduced to 10 −5 M. The XPS analysis (see Supplementary Fig. 6 ) indicates that the lower surface coverage obtained in these conditions increases the contribution of the higher energy contribution to the N 1s spectrum. On the basis of these evidences, the energy shift can be inferred to result either from stabilization effect of a cationic species formed during the grafting reaction by the silicon surface or from an electron depletion of the molecular system induced by the interaction with the surface, in analogy to similar effects experimentally observed and discussed for various phthalocyanine monolayers adsorbed on semiconducting oxides [41] , [42] , [43] but never reported for double-decker complexes. Density functional theory (DFT) calculations (see Supplementary Note 5 ) have been performed to clarify the effect of the oxidation of the double-decker systems on the XPS spectra as well as the perturbation caused by the silicon surface on the energy of core electrons in the complex. A non-periodic cluster approach, adopted to model the silicon surface, proved to be well suited in the perspective to obtain information on the core electron energy trend, even if a perfect reproduction of the experimental data is beyond the purposes of this paper. Results shown in Supplementary Fig. 7 evidence that nitrogen 1s electrons are dispersed around a single energy value in the neutral double-decker species in the gas phase. Similar findings emerge on the cationic species but the mean value is significantly shifted at higher energy (+2.4 eV) because of the effect of the positive charge on the core electron distribution. Once the double deckers lie in contact with the silicon surface, the nitrogen 1s electrons remain dispersed around a single energy value in both neutral and cationic species. A small energy shift (+0.1 eV) is observed on the neutral double decker, whereas a significant shift to lower binding energy is observed for the cationic species as a consequence of the ion pair formation between the positively charged molecule and negatively charged surface, where one oxo-termination has been introduced to respect the charge neutrality. This effect, however, decreases significantly by increasing the Si cluster size used to model the surface ( Supplementary Fig. 8 ), and an accurate estimation of the energy difference between neutral and cationic species on surface cannot be achieved. Nevertheless, these theoretical results confirm our assignement of the observed N 1s shift to electron-depleted TbPc 2 species stabilized by the silicon surface. Structural characterization of the TbPc 2 (OC 11 H 21 ) 8 @Si monolayer Linear and circular polarization-dependent X-ray absorption experiments have been carried out on the TbPc 2 (OC 11 H 21 ) 8 @Si monolayer to evaluate with the highest level of accuracy the structural and magnetic properties of the assembled nanostructure. Actually the element selectivity of this synchrotron-based technique guarantees addressing directly the properties of the anchored molecules by focusing the measurements at the Tb M 4,5 absorption edges, whereas the surface sensitivity is warranted by the adopted detection mode, that is, the Total Electron Yield (TEY) mode [44] . Moreover, the DEIMOS beamline, located at Synchrotron SOLEIL, has been specifically designed to carry such measurements: very high beam stability combined with reduced photon flux guarantee measurements reproducibility without damaging the samples [45] . At first, X-ray Natural Linear Dichroism (XNLD) has been measured for the M 4,5 Tb edges. The sample has been set so that the normal to the surface n and the X-ray propagation vector k lie in the horizontal plane with ( n , k )=60°. The cross-sections with horizontal linear polarization ( σ H ) and with vertical linear polarization ( σ V ) have been measured (see Fig. 4a and Supplementary Fig. 9 ). 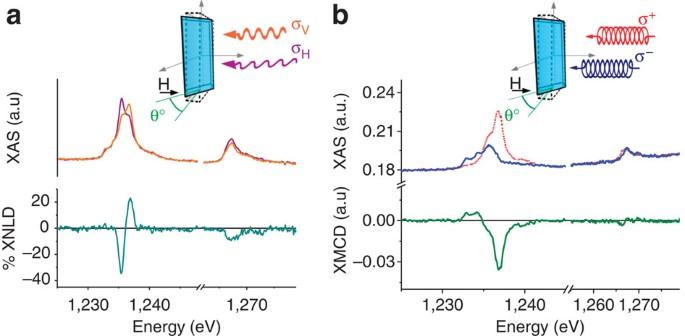Figure 4: X-ray polarized light absorption. XNLD (a) and XMCD (b) measurements at 2.2±0.2 K, 50 kOe, for (n,k)=60°. In the inset, the geometry of the two experiments are presented: in a XNLD experiment vertical (σV) and horizontally (σH) polarized light are used and the sample is rotated by an angleθbetween the normal to the surface and the X-ray light propagation direction, an external magnetic field is used only to enhance the TEY detection capabilities; in XMCD experiment, light with opposite circular polarization,σ+andσ−, is employed in an analogous experimental geometry, external magnetic field andθare varied to extract additional information. Figure 4: X-ray polarized light absorption. XNLD ( a ) and XMCD ( b ) measurements at 2.2±0.2 K, 50 kOe, for ( n , k )=60°. In the inset, the geometry of the two experiments are presented: in a XNLD experiment vertical ( σ V ) and horizontally ( σ H ) polarized light are used and the sample is rotated by an angle θ between the normal to the surface and the X-ray light propagation direction, an external magnetic field is used only to enhance the TEY detection capabilities; in XMCD experiment, light with opposite circular polarization, σ + and σ − , is employed in an analogous experimental geometry, external magnetic field and θ are varied to extract additional information. Full size image In the ideal case where TbPc 2 molecules adopt a lying down configuration, that is, the phthalocyaninato C 4 axis is parallel to the surface normal, the electric field of the vertically polarized light is aligned perpendicular to the symmetry axis of the coordination square antiprism of the Tb III ion, whereas the horizontal one forms an angle of 30° with this axis. In the opposite case, where TbPc 2 molecules adopt a standing configuration with no order in the plane, the electric field of the vertically polarized light can be now aligned at any angle with the symmetry axis of the molecules, whereas for the horizontal polarization, the electric field cannot be parallel to the molecular symmetry axis. It is thus straightforward that XNLD, evaluated as ( σ v − σ H ), changes sign for the two configurations and can therefore be employed to extract information on the molecular arrangement in the monolayer. By the comparison (see Supplementary Note 6 ) with experimental and theoretical reports from earlier literature [27] , it can be straightforwardly assessed that the molecules forming the monolayer are preferentially oriented with a lying down configurations, with the oriented molecules accounting for about half of the sample. It is interesting to notice that a reversed XNLD signal is measured in a bulk sample obtained by drop casting a solution of TbPc 2 (OC 11 H 21 ) 8 (see Supplementary Fig. 10 ). This finding is in line with the common tendency for thick bis(phthalocyaninato) films to aggregate in a standing up configuration [27] , and the observed difference between the two samples confirms that our monolayer of TbPc 2 does not contain physisorbed aggregates. Magnetic characterization of the TbPc 2 (OC 11 H 21 ) 8 @Si monolayer X-ray absorption experiments carried out at low temperature, under a 50-kOe magnetic field parallel to the X-ray light propagation vector, using circularly polarized light allowed to extract also the X-ray Magnetic Circular Dichroism (XMCD). This is defined as the difference ( σ − − σ + ) between the absorption spectra obtained with right ( σ − ) and left ( σ + ) polarized light. The result for the monolayer is reported in Fig. 4b : detected features and the intensity of the dichroic signal are in line with the expected ones [27] , [28] for a saturated Tb 3+ system characterized by total angular momentum J = L+S =6. 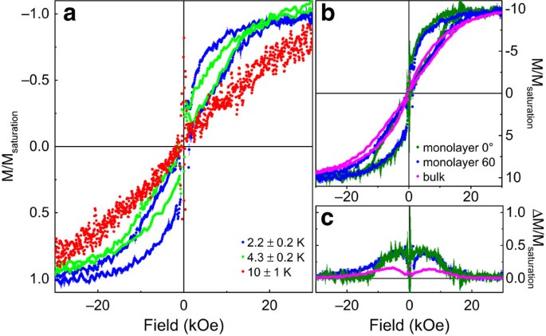Figure 5: TbPc2(OC11H21)8@Si hysteresis. (a) XMCD-detected magnetization curves for (n,k)=60° as a function of the temperature in the TbPc2(OC11H21)8@Si monolayer. (b,c) Comparison between the behaviour of the thick film and the monolayer, the latter being measured for (n,k)=0° and 60°. These magnetization curves, measured in the same condition for all the samples (2.2±0.2 K and 500 Oe s−1scan speed) through the XMCD technique, are reported inbwith their experimental error. Inc, the hysteresis opening is estimated as ΔM(H) according to the procedure described in the text. Figure 5a reports the variation of the XMCD contribution at the M 5 edge, normalized to the saturation value, as a function of the applied magnetic field between −50 and 50 kOe at three different temperatures. We stress here that, profiting from the fast TEY detection setup and the stability of the experimental apparatus developed in the DEIMOS beamline [45] , it has been possible to collect the signal as a function of the fast sweeping field, thus providing highly resolved XMCD-detected magnetization curves clearly showing hysteretic behaviour already at 4.3±0.2 K. Figure 5: TbPc 2 (OC 11 H 21 ) 8 @Si hysteresis. ( a ) XMCD-detected magnetization curves for ( n , k )=60° as a function of the temperature in the TbPc 2 (OC 11 H 21 ) 8 @Si monolayer. ( b , c ) Comparison between the behaviour of the thick film and the monolayer, the latter being measured for ( n , k )=0° and 60°. These magnetization curves, measured in the same condition for all the samples (2.2±0.2 K and 500 Oe s −1 scan speed) through the XMCD technique, are reported in b with their experimental error. In c , the hysteresis opening is estimated as Δ M ( H ) according to the procedure described in the text. Full size image The opening of the hysteresis strongly depends on the temperature and also on the speed of the scanning field (see Supplementary Fig. 11 ), confirming the dynamic character of the magnetic bistability typical of TbPc 2 SMMs. A tiny angular dependence of the hysteresis is also detected (see Fig. 5b and Supplementary Fig. 11 ) in line with the XNLD indications of a partial orientation of the molecular film. Most important is that the comparison with the behaviour of the bulk phase (see Fig. 2c , and Supplementary Fig. 12 for a direct comparison at the same field scan rate) reveals a significantly larger opening of the hysteresis for the monolayer. To further investigate this aspect, an analogous XMCD characterization has been carried out on the drop cast thick film of TbPc 2 (OC 11 H 21 ) 8 , evidencing an opening on the hysteresis cycle significantly weaker than in the monolayer grafted to the Si surface (see Fig. 5b ), in line with standard magnetometry experiments on the pristine compound. A better estimation of the changes in the hysteretic behaviour can be achieved by plotting the difference in the magnetization obtained for increasing and decreasing field: Δ M ( H )=| M ( H ↑)− M ( H ↓)| The area under these curves ( Fig. 5c ) thus corresponds to the opening of the hysteresis loop, which results to be significantly larger in the monolayer sample than in the thick film. A similar enhancement of the bistable behaviour in the monolayer is also observed for hysteresis curves taken at different orientation of the substrate in respect to the magnetic field ( Fig. 5 and Supplementary Fig. 11 for more data), thus indicating that the observed phenomenon is not due to orientation effects but has to be related to the grafting process. The profusion of experiments performed on the TbPc 2 family of SMM has revealed significant changes in the magnetic bistability depending on the nature of the substrate the SMM is deposited onto. The mechanism of these modifications remains, however, obscure. With metallic substrates, the typical butterfly hysteresis observable well above helium temperature disappears, although pyrene-functionalized TbPc 2 when grafted to single-wall carbon nanotubes exhibits an increase of the remnant magnetization at sub-kelvin temperatures [46] that is the opposite of the trend observed when other SMM are grafted to carbon nanotubes [47] . When ferromagnetic substrates are employed, the TbPc 2 hysteresis is observed at much higher temperatures [29] but the bistability and coercivity are those of the substrate and cannot be considered an intrinsic property of the single molecule. We notice that an enhancement of the opening of the hysteresis has been observed [40] at 1.5 K in frozen solution by oxidation of the double decker to the cationic [TbPc 2 ] + species, an effect that seems further enhanced in the monolayer investigated here. The use of silicon, unprecedented for this type of SMMs, presents several interesting advantages. Our results show that TbPc 2 SMMs can be covalently and robustly anchored to a silicon substrate, with the deposited monolayer standing harsh treatments like sonication in dichloromethane. Si–C covalent bonds in fact guarantee a higher stability respect to π-stacking or S–Au interactions. Moreover, the pronounced magnetic bistability not only is retained at the level of the monolayer but, when quantified as the area enclosed in the hysteresis cycle, it happens to be significantly enhanced by the grafting process to silicon, even if with small remnant magnetization. More important is that this alteration correlates with changes observed in the photoelectron spectra. Although the long alkyl chains in this Tb double-decker SMM could in principle hamper a significant interaction with the substrate, their flexibility, as already observed for functionalized TbPc 2 molecules grafted on gold [48] , induces a preferential lying down configuration that can allow a stabilization of an oxidized TbPc 2 system by the silicon substrate as indicated by coverage-dependent XPS results. It is well known that the oxidation of the Pc ligands reduces the height of the square-antiprism coordination polyhedron with a sensible enhancement of the effective energy barrier for the reversal of the magnetization and more pronounced hysteretic behaviour [15] , [16] , [49] . Covalent grafting to the silicon surface appears to have a similar effect on the electron density of the phthalocyanine rings and is therefore not unreasonable that it can equally affect the magnetic anisotropy of the complex, enhancing the magnetic bistability, although not preventing tunnelling in zero field. In conclusion, our XMCD observation of the enhanced magnetic hysteresis evidences that a careful choice of the substrate and of the grafting strategy can be exploited to tune the electronic properties of these SMMs and optimize their magnetic behaviour, in contrast to what has been observed by assembling the pristine TbPc 2 system on solid surfaces by thermal evaporation procedures in UHV [27] , [29] , [30] , [50] , [51] . The chemical robustness of these covalently grafted monolayers make them suitable for insertion in spintronic devices prepared by solution techniques, which is the emerging trend in this rapidly evolving field [52] . Synthesis of TbPc 2 (OC 11 H 21 ) 8 To a stirred solution of 4-(ω-undecenyloxy)phthalonitrile ( 2 ) (400.0 mg, 1.35 mmol, see Supplementary Note 1 ) in 1-hexanol (8 ml) [Tb(acac) 3 ]· n H 2 O (98.6 mg, 0.216 mmol, 0.16 equiv) was added followed by 1,8-Diazabicyclo[5.4.0]undec-7-ene (202.0 μl, 1.35 mmol, 1 equiv). The reaction was heated to reflux and stirred for 16 h. The dark-green mixture was cooled to room temperature and the solvent removed under reduced pressure. Methanol was added to the residue until a precipitate formed. The green finely dispersed mixture was filtered off and purified by flash chromatography (CHCl 3 as eluent) to obtain a green solid (149.2 mg, 35% yield). Ultraviolet–visible: λ max (CHCl 3 ) 926, 681, 469, 361, 329 nm; MALDI-TOF: [M] + calculated for C 152 H 192 N 16 O 8 Tb=2,529.439 m / z ; found=2,529.444 m / z . Magnetic characterization of the bulk system Quantum Design PPMS Vibrating Sample Magnetometer (Quantum Design) setup in the continuous measurement mode sweeping the magnetic field at 50 Oe s −1 was used to characterize a bulk TbPc 2 (OC 11 H 21 ) 8 sample, pressed in a pellet, between −50 and 50 kOe. AC magnetic susceptibility up to 10 kHz of this sample was measured with the same Quantum Design PPMS platform in zero and 5 kOe static fields. Quantum Design MPMS SQUID magnetometer was employed to extend the AC susceptibility measurements in the low-frequency range (down to 0.1 Hz). Monolayer preparation The TbPc 2 (OC 11 H 21 ) 8 solution in mesitylene were placed in a small, three-necked flask fitted with a nitrogen inlet and a condenser. The solutions were deoxygenated with dry nitrogen for at least 1 h. Subsequently, p -doped Si(100) (Boron doped, resistivity 1.5–4 Ω cm) substrates were treated in a piranha solution for 12 min, rinsed in water for 2 min, and etched in 1.0% hydrofluoric acid for 90 s, then immediately placed in the alkenes solution. The solutions were then refluxed at 200 °C for 2 h, under slow N 2 bubbling to prevent bumping. After cooling to RT, the samples were removed from the flask and cleaned by several rinsing cycles of ultrasonic cleaner. XPS measurements XPS spectra of the monolayer of TbPc 2 (OC 11 H 21 ) 8 @Si were run with a PHI 5600 multitechnique ESCA-Auger spectrometer equipped with a monochromatic Al Kα X-ray source. Analyses were carried out with an analyser pass energy of 23.5 eV and a photoelectron angle of 45° (relative to the sample surface) with an acceptance angle of ±7°. Bulk drop cast and Cl 2 -treated TbPc 2 (OC 11 H 21 ) 8 sample have been measured with a VSW setup equipped with non-monochromatic Al Kα source not focalized; in this case the angle between the analyser axis and the X-ray propagation vector from the X-ray source was 54.44° and a pass energy of 44 eV was used. These different conditions were required to properly characterize these samples avoiding the reduction of the oxidized system by the effect of the photo-electrons and secondary electrons. In all spectra, XPS-binding energy scale was calibrated by placing the C 1s peak due to hydrocarbon moieties and ‘adventitious’ carbon at 285.0 eV. Data analysis was performed using a mixed Gaussian and Lorentzian line-shape and background subtraction using a Shirley function. The elemental composition of the samples was evaluated by estimating the integrated area of each component corrected for the corresponding photo-ionization cross-section [53] . The Tb 3d 3/2 sensitivity factor was empirically verified from terbium(III)acetate hydrate powder (see Supplementary Fig. 13 ). X-ray absorption spectroscopy measurements X-ray absorption spectroscopy (XAS) and XMCD spectra at the Tb M 4,5 edges were recorded at the DEIMOS beamline [44] , Synchrotron SOLEIL facility in France, on a UHV compatible pumped 4 He cryo-magnet. Absorption spectra were measured in TEY detection mode to guarantee the optimal detection sensitivity. All the characterizations were performed using a low density of photons to avoid radiation damages. XNLD experiments were carried out by recording XAS with linearly polarized light (vertical and horizontal polarization) in a 50-kOe field (to enhance the TEY) placing the normal of sample surface at 60° with respect to the X-ray light propagation vector and extracted as ( σ V - σ H ). Final XNLD spectrum is the result of the averaging of four scans per polarization, for both positive and negative magnetic field in order to avoid contamination from spurious X-ray Magnetic Linear Dichroism (XMLD) signal. XMCD spectra were obtained with a similar averaging procedure [54] from circularly polarized (left and right) absorption spectra measured at the temperature of 2 K and under an applied magnetic field of 50 kOe parallel to the X-ray propagation vector. The same setup was used to record the XMCD dependence on the magnetic field (hysteresis curves) as a function of sample orientation and temperature, as well as field sweeping rate. Data have been normalized with respect to the saturation value in order to be able to compare this experiment with traditional magnetometry experiments and evaluate the angular dependence. DFT calculations Calculations were performed adopting the Perdew, Burke and Ernzerhof (PBE) formalism for both exchange and correlation functionals [55] . The effective core potential of Hay and Wadt [56] was used for the yttrium and terbium atoms. The standard all-electron 6–31G** basis was used for all remaining atoms [57] . Closed or open shell approach are adopted depending on the charge state of the double-decker system we considered: for a +1 charged system a closed shell is adopted, whereas for the neutral bis-phthalocyaninato system an open shell is adopted to take into account the electron multiplicity. Si(100) surface was represented by a cluster of 21 silicon atoms H-terminated with one hydroxyl termination. Moving from the gas phase to the surface-absorbed molecules, TbPc 2 was replaced by YPc 2 to avoid convergence complication due to the high multiplicity arising from f electrons of the terbium atom (see Supplementary Note 5 for further details). Molecular geometry optimization of stationary points was carried out without symmetry constrains and was based on an analytical gradient minimization approach. All calculations were performed using NWCHEM code [58] on Linux cluster systems. How to cite this article: Mannini, M. et al . Magnetic behaviour of TbPc 2 single-molecule magnets chemically grafted on silicon surface. Nat. Commun. 5:4582 doi: 10.1038/ncomms5582 (2014).